Self-templated chemically stable hollow spherical covalent organic framework Covalent organic frameworks are a family of crystalline porous materials with promising applications. Although active research on the design and synthesis of covalent organic frameworks has been ongoing for almost a decade, the mechanisms of formation of covalent organic frameworks crystallites remain poorly understood. Here we report the synthesis of a hollow spherical covalent organic framework with mesoporous walls in a single-step template-free method. A detailed time-dependent study of hollow sphere formation reveals that an inside-out Ostwald ripening process is responsible for the hollow sphere formation. The synthesized covalent organic framework hollow spheres are highly porous (surface area ∼ 1,500 m 2 g −1 ), crystalline and chemically stable, due to the presence of strong intramolecular hydrogen bonding. These mesoporous hollow sphere covalent organic frameworks are used for a trypsin immobilization study, which shows an uptake of 15.5 μmol g −1 of trypsin. Covalent organic frameworks (COFs) represent a new family of crystalline porous materials, with a well-defined and predictable network of molecular building blocks [1] . These materials showcase promising applications in the field of gas storage [2] , [3] , [4] , [5] , opto-electronics [6] , catalysis [7] , [8] , [9] and sensing [10] because of their crystalline and periodic structure with high surface area and thermal stability. COFs are usually synthesized as microcrystalline powders and their long-range growth is limited in the nano/micro domain due to the internal defects [11] , [12] , [13] . COF crystallites have been reported to have adopted various shapes such as belts [6] , fibres [14] , sheets [15] , cubes [16] , rectangular prisms [17] , spheres and platelets [18] . However, the mechanisms of the formation and self-assembly of COF crystallites are still poorly understood. The shape of a crystallite is an extremely important factor in molecular absorption and catalysis [19] , [20] . In this regard, hollow spherical structures are considered to be an important morphology because of their potential application in catalysis [21] , [22] , [23] , [24] , drug delivery [25] , molecular sensors and in energy storage [26] . Although active research on the design and synthesis of COFs has been ongoing for almost a decade, there has been only one report of a COF with hollow spherical morphology without much structural (because of poor crystallinity) and mechanistic insight of the hollow sphere formation [27] . Moreover, the mixed morphology of the sheets and spheres reported to be found in the reaction medium make the isolation of pure hollow spheres extremely difficult and the chemical instability makes this hollow spherical COF inefficient for any practical use. Herein, we report the synthesis of a chemically stable hollow spherical COF ( DhaTab ) with high surface area ( ∼ 1,500 m 2 g −1 ) mesoporous walls and chemical stability via self-templated synthesis. Furthermore, we also report the mechanism of the hollow sphere formation of crystalline COF in detail using different microscopic techniques. Self-templated synthetic methods [28] , [29] , [30] , [31] , [32] , [33] , [34] , [35] are considered to be the most cost-effective synthetic methods for hollow sphere synthesis, since they do not require sacrificial templates. Template-free methods also avoid problems such as shell collapse and pore contamination during template removal [33] , [34] , [35] . Although self-templating has been the major recipe for the synthesis of metal oxide and metal sulfide-based hollow spheres [32] , [33] , [34] , this method has been less explored to synthesize organic and polymer-based hollow spheres [35] , [36] , [37] . The hollow spherical COF ( DhaTab ), reported in this paper, consists of a macroporous inner cavity (pore width 0.5–2 μm) wrapped up by the mesoporous COF shell (width 20–40 nm). It is noteworthy that the application of COFs is still mostly limited to the storage of gas molecules, since most of the COFs synthesized are microporous in nature and their pores are not sizable enough to hold larger guests, such as enzymes [38] , [39] , [40] . While examples of mesoporous boronic acid-based COFs have been reported in the literature [41] , [42] their chemical instability prevents the usage of these materials for the storage of drugs and enzymes [43] , [44] . Since the COF- DhaTab is chemically stable and mesoporous (3.7 nm), we can study the adsorption and storage of the enzyme trypsin into the COF pores. Immobilization of enzyme into the mesoporous material is potentially useful for applications such as biosensors and biocatalysts because it can increase the recyclability of the costly enzyme and also improves the stability of enzymes under extreme conditions [45] , [46] , [47] , [48] . Synthesis and characterization Synthesis of COF- DhaTab and DhaBad was carried out by the Schiff base reaction between 2,5-dihydroxyterephthalaldehyde ( Dha ; 21.6 mg) and 1,3,5-tris(4-aminophenyl)benzene ( Tab ; 30.2 mg) or N 1 ,N 1 -bis(4-aminophenyl)benzene-1,4-diamine ( Bad ; 26.1 mg) in mesitylene-dioxane (1.7 ml:0.3 ml) solvent combination and a catalytic amount of 0.2 ml (8 M) acetic acid. A yellow and red-coloured fluffy powder of DhaTab and DhaBad were collected by centrifugation or filtration and washed with dimethylacetamide (DMAc), water and ethanol. The synthesis of the hollow spherical COF was carried out in a single-step Schiff base reaction without using any template. Self-templated hollow sphere formation happens mainly because of the Kirkendall [29] , [30] , [31] , [32] effect and Ostwald ripening [34] , [35] . Among them, Ostwald ripening was proved to be the main reason for the formation of metal oxide and sulphide-based hollow spheres [34] , [35] . Rods like crystallites of COF- DhaTab were formed initially in 12 h and these crystallites randomly self-assembled into coiled or dense spheres. Since the crystallites in the inner part of the sphere have got higher surface energy than those on the outer surface [21] , an inside-out Ostwald ripening happened after 24 h and hollow spheres of COF- DhaTab were formed. As the time progresses, crystallites on the sphere wall fused together to produce a smooth surface. These hollow spheres are highly porous, crystalline, chemically stable and can retain their spherical morphology in water and phosphate buffer. The chemical stability and high surface area of the COF -DhaTab arises because of the strong intramolecular hydrogen bonding that locks the phenyl rings in one plane and protects the imine nitrogen from nucleophilic attack [49] , [50] , [51] , [52] . Fourier transform infrared (FT-IR) spectra of COF- DhaTab indicates the total consumption of the starting material, as the characteristic –C=O (1,662 cm −1 ) stretching band of Dha and –N-H ( ∼ 3,300 cm −1 ) stretching band of Tab were absent ( Supplementary Fig. 1 ). The formation of the imine bond can be understood from the FT-IR peak at 1,613 cm −1 , which corresponds to the –C=N stretching and the value appears near to the –C=N stretching band of the monomer unit at 1,617 cm −1 ( Fig. 1c ). Similarly, DhaBad shows the imine bond (–C=N) stretching at 1,607 cm −1 , which is close to 1,611 cm −1 , the –C=N stretching value of the monomer ( Supplementary Figs 2 and 3 ). The imine bond formation and the existence of COF as the enol form was confirmed from the 13 C CP-MAS solid-state nuclear magnetic resonance (NMR) spectrum of COF- DhaTab and the corresponding monomer unit ( Fig. 1d ). These 13 C CP-MAS data show similar location of the imine carbon peak of the COF at 155 p.p.m. with respect to the imine carbon peak of the monomer unit (152 p.p.m.). Scanning electron microscopy (SEM), transmission electron microscopy (TEM) and atomic force microscopy (AFM) were used to explore the morphology of the COF- DhaTab particles. SEM images show that DhaTab comprises a large number of interconnected hollow spherical particles with an average diameter of 0.5–4 μm ( Fig. 2a and Supplementary Fig. 4 ). Broken walls of some of the spheres (resulted during sonication) showcase the hollow interior cavity ( Fig. 2a ). TEM images of the hollow spherical COF- DhaTab showcase a bright area at the centre of each sphere and a dark contrast at the sphere wall, which is one of the main characteristic features of the hollow spheres ( Fig. 2b and Supplementary Fig. 5 ). However, the thickness of the sphere wall is not constant, and varies from 40 to 80 nm. On the other hand, SEM images of the DhaBad show the morphology of giant hollow spheres, which is formed by the self-assembly of small spheres. From the TEM images it was understood that the smaller spheres are also hollow in nature ( Supplementary Figs 6 and 7 ). The spherical morphology of COF- DhaTab particles was further understood from the AFM images, which shows that the surface of the hollow sphere is smooth. However, the cross-section analysis revealed that the diameters of the hollow spheres are in the range of 0.5–3 μm and the height was measured in the range of 100–150 nm ( Supplementary Figs 8 and 9 ). This large diameter-to-height ratio also indicates the hollow nature of the spheres. Since the sphere walls are made up of soft organic material, the high local force applied by the AFM tip flattened these hollow spheres. We have observed some donut-shaped objects while doing the AFM imaging, which supports this flattening of the hollow spheres ( Supplementary Fig. 9 ). This was due to the deformation of the hollow spheres under the influence of the AFM tip [28] . Thermal stability of the COF- DhaTab and DhaBad hollow spheres was monitored by Thermogravimetric analysis (TGA) under N 2 atmosphere. The COF- DhaTab framework was found to be stable up to 350 °C without much weight loss. The sharp weight loss (45%) observed after 400 °C was due to the decomposition of the framework ( Supplementary Fig. 10 ), while DhaBad hollow spheres show thermal stability up to 400 °C ( Supplementary Fig. 11 ). 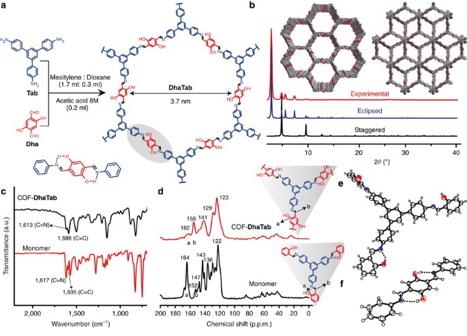Figure 1: Synthesis and characterization of COF-DhaTab. (a) Synthesis of COF-DhaTabby the Schiff base reaction ofTabandDha. (b) The experimental PXRD pattern ofDhaTab(red) compared with simulated eclipsed (blue) and staggered (black). (c) Comparison of FT-IR spectra ofDhaTab(black) with the monomer (red). (d) Comparison of solid-state13C NMR spectra ofDhaTab(red) with the monomer (black). (e) Oak Ridge thermal-ellipsoid plot (ORTEP) diagram ofDhaTabtriphenyl core monomer unit (2,2'-[[5'-[4-[[(2-hydroxy-phenyl)methylene]amino]phenyl] [1,1':3',1''-terphen-yl]-4,4''-diyl]bis (nitrilomethy-lidyne)]). (f) ORTEP diagram ofDhaTablinker unit (2,5-bis((E)-(phenylimino)methyl)benzene-1,4-diol). Figure 1: Synthesis and characterization of COF-DhaTab. ( a ) Synthesis of COF- DhaTab by the Schiff base reaction of Tab and Dha . ( b ) The experimental PXRD pattern of DhaTab (red) compared with simulated eclipsed (blue) and staggered (black). ( c ) Comparison of FT-IR spectra of DhaTab (black) with the monomer (red). ( d ) Comparison of solid-state 13 C NMR spectra of DhaTab (red) with the monomer (black). ( e ) Oak Ridge thermal-ellipsoid plot (ORTEP) diagram of DhaTab triphenyl core monomer unit (2,2'-[[5'-[4-[[(2-hydroxy-phenyl)methylene]amino]phenyl] [1,1':3',1''-terphen-yl]-4,4''-diyl]bis (nitrilomethy-lidyne)]). ( f ) ORTEP diagram of DhaTab linker unit (2,5-bis((E)-(phenylimino)methyl)benzene-1,4-diol). 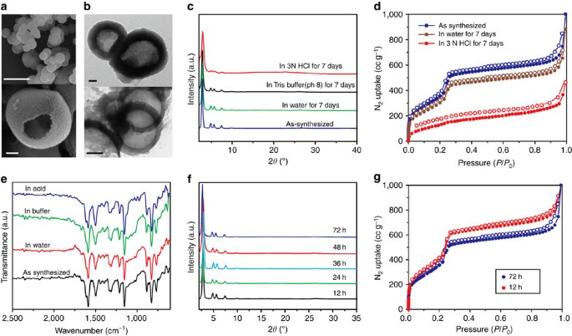Figure 2: Stability- and time-dependent structural characterization of COF-DhaTab. (a) SEM images of COF-DhaTabhollow spheres. (b) Transmission electron microscopy (TEM) images of COF-DhaTabhollow spheres. (c) PXRD pattern showing the stability ofDhaTab. (d) N2sorption isotherms recorded forDhaTabbefore (blue) and after water treatment (wine), acid treatment (red) study. (e) FT-IR showing the chemical stability ofDhaTab. (f) PXRD ofDhaTabsynthesized at different intervals of time. (g) N2sorption isotherms recorded forDhaTabsynthesized at 12 h (red) and 72 h (blue) intervals of time. Scale bars, (a) 4 μm and 500 nm, (b) 100 and 200 nm. Full size image Figure 2: Stability- and time-dependent structural characterization of COF-DhaTab. ( a ) SEM images of COF- DhaTab hollow spheres. ( b ) Transmission electron microscopy (TEM) images of COF- DhaTab hollow spheres. ( c ) PXRD pattern showing the stability of DhaTab . ( d ) N 2 sorption isotherms recorded for DhaTab before (blue) and after water treatment (wine), acid treatment (red) study. ( e ) FT-IR showing the chemical stability of DhaTab . ( f ) PXRD of DhaTab synthesized at different intervals of time. ( g ) N 2 sorption isotherms recorded for DhaTab synthesized at 12 h (red) and 72 h (blue) intervals of time. Scale bars, ( a ) 4 μm and 500 nm, ( b ) 100 and 200 nm. Full size image Crystallinity and structural determination The high crystallinity of COF- DhaTab was revealed from the Powder X-ray diffraction (PXRD) analysis, as it shows an intense peak at 2.8° 2 θ (intensity ∼ 150,000 cps), which corresponds to the 100 plane. The other minor peaks were observed at 4.9, 5.6, 7.4, 9.8, 26.3° 2 θ in the PXRD pattern, corresponding to 110, 200, 120, 220 and 001 planes, respectively ( Fig. 1b ). The π–π stacking distances between the vertically stacked sheets were calculated to be ∼ 3.4 Å from the d spacing of the 001 plane. The high crystallinity of COF- DhaTab is due to the presence of intramolecular O−H···N=C hydrogen bonding between the hydroxyl and imine functional groups, which locks the phenyl rings in one plane and improves the stacking interaction between the adjacent COF layers ( Fig. 1a ). This improved structural rigidity and planarity of the framework, together with the all trans -conformation of the imine bond, results in the increase in the crystallinity of COF- DhaTab . In order to understand the effect of H-bonding within the COF architecture, we have crystallized the monomer units 2,2′-[[5′-[4-[[(2-hydroxyphenyl)methylene]amino]phenyl][1,1′:3′,1″-terphen-yl]-4,4″-diyl]bis(nitrilomethylid-yne)] and 2,5-bis((E)-(phenylimino)methyl)-benzene-1,4-diol ( Fig. 1e,f , Supplementary Figs 12 and 13 and Supplementary Data 1 ) of the COF- DhaTab . The crystal structural determination of the monomer units reveals that the central triphenyl core in COF- DhaTab is not in the same plane as reported for the COF-8 (ref. 53 ), COF-43 (ref. 54 ) and BTP-COF [55] . The phenyl rings within the monomer units are a little tilted with respect to the central benzene ring in order to avoid the steric repulsion between the hydrogen atoms ( Fig. 1e ). However, the monomer unit that connects one triphenyl core to another to construct the framework ( Fig. 1f ) is perfectly planar with almost zero dihedral angle ( θ =0.82° and θ =0.05°) between the central and the end phenyl rings. This planarity arises because of the strong intramolecular O−H···N=C H-bonding [56] , [57] , [58] , [59] , [60] ( D =2.619(2) Å, d =1.895(2) Å, θ =146.68° (3)) as well as continuous conjugation. A possible eclipsed two-dimensional (2D) model for the COF- DhaTab was built using Materials Studio version 6.1, in order to find out the structure and the unit cell parameters. The modelling of COF- DhaTab cannot be carried out in the conventional P 6/ m space group since the central triphenyl system is not planar. Hence, we decided to model COF- DhaTab in the P 3 space group, with the unit cell parameters a = b =36.2 Å, c =3.4 Å and α = β =90°, γ =120° ( Supplementary Figs 14 and 15 , Supplementary Table 1 ). Pawley refinement was performed using the Reflex Plus module of Materials Studio, which showcases good agreement between simulated and experimental PXRD patterns (R-pattern factor (Rp)=2.5%, R-weighted-profile factor (Rwp)=4.5%; Supplementary Fig. 16 ). We have further modelled the staggered structure of COF- DhaTab in R 3 space group with the unit cell parameter a = b =36.2 Å, c =10 Å and α = β =90°, γ =120° ( Supplementary Fig. 17 , Supplementary Table 2 ). However, the simulated PXRD pattern for the staggered conformation has poor matching (Rp=70.5%, Rwp=78%) with the experimental PXRD pattern ( Supplementary Fig. 18 ). We have observed that as compared with COF- DhaTab , the crystallinity of DhaBad is very poor ( Supplementary Fig. 19 ). The non-planarity of the phenyl rings was not the reason for the low crystallinity [61] . We have synthesized and crystallized the monomer of DhaBad to find out the reason for this anomaly. From the single crystal data it was evident that the monomer of DhaBad contains two imine bonds in same direction, and it is not C 3 -symmetric ( Supplementary Fig. 20 ). Since the monomer of DhaBad does not obey the basic criteria of symmetry to form the hexagonal COF, it is impossible to construct a closed hexagonal pore and an extended ordered structure, with a non-C 3 -symmetric COF building block [62] . Gas adsorption The N 2 adsorption was carried out for the activated COF- DhaTab sample in order to evaluate the permanent porosity. COF- DhaTab exhibits reversible type IV isotherm, which is one of the main characteristics of mesoporous materials. The surface area of COF- DhaTab was calculated to be 1,480 m 2 g −1 using the Brunauer–Emmett–Teller (BET) model ( Fig. 2d and Supplementary Fig. 21 ). The high surface area of COF- DhaTab as compared with its non-hydroxyl analogue MOP (A-B1) [63] was due to the presence of strong intramolecular H-bonding, which imparts structural rigidity to the material and also improves the planarity of the 2D layers( Supplementary Fig. 22 ). This can be understood from the single crystal data of the monomer ( Fig. 1f and Supplementary Fig. 8 ), which shows that the three phenyl rings lie in one plane. The improved planarity and structural rigidity will help in arranging the COF layers in an ordered way, which will lead to an improvement in crystallinity and surface area. The pore size distribution of COF- DhaTab was calculated using the Barrett–Joyner–Halenda desorption model, which shows peak maxima at 3.7 nm, which is very close to the theoretically predicted value (3.6 nm) ( Supplementary Fig. 23 ). COF- DhaTab shows moderate H 2 and CO 2 uptake capacity, which was calculated to be 120 cm 3 g −1 (77 K) and 78 cm 3 g −1 (273 K) at 1 bar pressure ( Supplementary Figs 24 and 25 ). Surface area of DhaBad was also calculated using the BET method, which shows a moderate value of 447 m 2 g −1 ( Supplementary Fig. 26 ). The low surface area of DhaBad as compared with DhaTab was due to its disordered structure. Chemical stability The chemical stability of the hollow spherical COF -DhaTab in water was investigated by submerging the 30 mg of material in 10 ml water for 7 days. Retention of peaks in the PXRD pattern and non-alteration of the FT-IR peaks after the water treatment shows the structural rigidity of this material in water ( Fig. 2c,e ). N 2 adsorption isotherms show that COF- DhaTab remains porous even after prolonged water treatment with a small decrease in the surface area (1,480 versus 1,220 m 2 g −1 ; Fig. 2d ). In addition to that, we have performed water vapour adsorption studies of COF- DhaTab , which shows reversible water vapour uptake and confirms the stability of COF in water ( Supplementary Fig. 27 ). In addition to this, elemental analysis of the COF sample was performed before and after the water stability test. 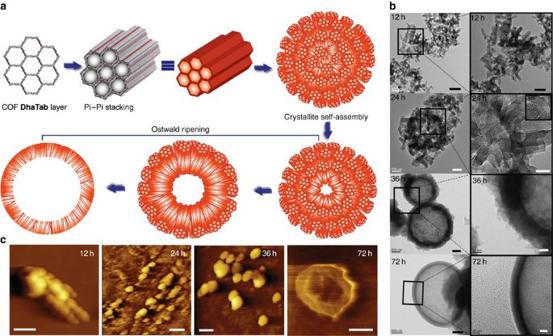Figure 3: Mechanism of hollow sphere formation. (a) Proposed mechanism of the formation of COF hollow spheres. (b,c) TEM and AFM images of COF-DhaTab, respectively, recorded at different intervals of time. Scale bars, (b) 12 h (200 nm, 100 nm), 24 h (100 nm, 50 nm), 36 h (200 nm, 50 nm), 72 h (200 nm, 20 nm) and (c) 12 h (500 nm), 24 h (500 nm), 36 h (100 nm), 72 h (100 nm). It was observed that the elemental weight percentage remains almost identical after the water treatment, which indicates the hydrolytic stability of the material ( Supplementary Table 3 ). To check the chemical stability in acid, a similar type of stability experiment was performed with 3 N HCl for 7 days. PXRD of the recovered COF- DhaTab samples after this acid treatment shows retention of all the main peaks, which indicates the retention of the framework structure in the acid-treated sample ( Fig. 2c and Supplementary Fig. 28 ). However, a decrease in surface area was observed, which may be because of protonation of the imine nitrogen ( Fig. 2d ). The protonation of the imine bond can be understood from the FT-IR spectra. In FT-IR it was seen that on treatment of COF- DhaTab with hydrochloric acid a new band arises at 1,646 cm −1 , which indicates the protonation of imine bond (1,645 cm −1 in monomer; Supplementary Fig. 29 ). The single crystal data of the protonated Schiff base compound o-(Salicylideneamino) phenol shows that imine bonds are susceptible to protonation on treatment with hydrochloric acid ( Supplementary Fig. 30 ). [64] 1 H NMR studies of the monomer shows that there is a shift in the position of the –OH proton on hydrochloric acid treatment. This can be because of the loss of intramolecular hydrogen bonds up on protonation of imine bonds ( Supplementary Fig. 29 ). Additional stability experiments were performed in a phosphate buffer of pH 7.4, since the enzyme encapsulation studies were later performed in the buffer media. Retention of PXRD peaks and unchanged morphology observed from the TEM images confirms the stability of COF- DhaTab in phosphate buffer media ( Fig. 2c ). In addition to this, we have checked the hydrothermal stability of COF-DhaTab at different temperatures (40, 60 and 80 °C) for 24 h. The unaltered PXRD and FT-IR patterns confirm the hydrothermal stability of the material ( Supplementary Fig. 28 ). COF- DhaTab was found to be unstable under basic conditions ( 3 N NaOH; Supplementary Fig. 31 ). The chemical stability of COF- DhaTab was due to the presence of the intramolecular O-H···N=C hydrogen bonding, which protects the imine bond from the attack of the nucleophiles [48] , [49] , [50] , [51] . Treatment with NaOH will cause the removal of the phenolic (−OH) hydrogen, which is responsible for hydrogen bonding ( Supplementary Fig. 32 ). Absence of this intramolecular O-H···N=C hydrogen bonding and the presence of Na + ion near to the phenolate anion present in different COF layers disturb the ordered layer stacking, which may cause the disintegration of COF- DhaTab hollow spheres. To prove this we have performed the dynamic light-scattering study of the leached out sample, which shows the presence of particle having size less than 10 nm, which is very small as compared with the size of the COF hollow spheres ( Supplementary Fig. 33 ). SEM imaging of the COF- DhaTab sample before and after treatment shows that the hollow sphere morphology of the COF- DhaTab was lost after the base treatment and the morphology transforms into aggregated platelet-like structure ( Supplementary Fig. 33 ). These results indicate that the hollow sphere morphology of COF- DhaTab gets disintegrated into small particles in the presence of NaOH, which may be the reason for the loss of crystallinity of DhaTab during NaOH treatment. Mechanism of hollow sphere formation We have studied the synthesis and morphological changes in COF- DhaTab at different time intervals (12, 24, 36, 48 and 72 h). COF- DhaTab synthesis was quenched by removing the reaction tubes from the oven at those specific time intervals. 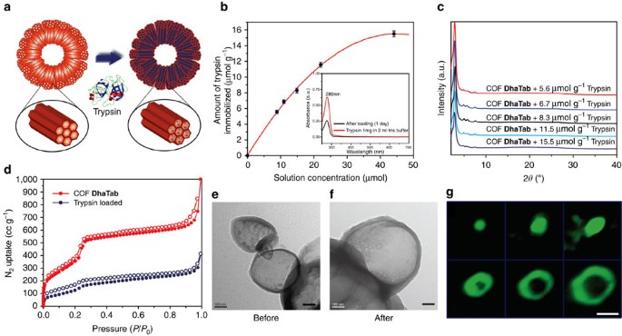Figure 4: Trypsin loading in COF-DhaTab. (a) Schematic representation of trypsin adsorption in COF-DhaTab. (b) Amount of trypsin loading in COF-DhaTabat different solution concentration (the error bars represent the s.d. from triplicate measurements). (c) PXRD patterns of DhaTab after the adsorption of trypsin. (d) Comparison of N2adsorption isothermsDhaTabbefore and after trypsin loading. (e) TEM image ofDhaTab(e) before and (f) after enzyme adsorption. (g) Confocal Z stacks of sections of fluorescein-labelled trysin-loaded single COF-DhaTab hollow sphere. Scale bars, (e) 100 nm, (f) 100 nm and (g) 2 μm. Furthermore, we have analysed the COF- DhaTab samples isolated after 12-, 24-, 36-, 48- and 72-h reaction time using FT-IR, NMR, TGA, PXRD, N 2 adsorption and elemental analysis ( Supplementary Table 4 ). Identical PXRD patterns of the COF- DhaTab samples synthesized at different time intervals (12, 24, 36, 48 and 72 h; Fig. 2f ) indicate that COF crystallite formation is complete even at shorter reaction time ( Fig. 2f ) [65] , [66] . COF -DhaTab samples synthesized at shorter reaction time (12 h) also show identical FT-IR, 13 C CP-MAS and N 2 adsorption isotherm (1,536 and 1,480 m 2 g −1 ), which is an extremely important observation and rarely studied in COFs ( Fig. 2g ) [65] , [66] . Our observation indicates that the large-scale synthesis of good-quality COFs is possible in a shorter reaction time, just like its inorganic counterpart MOFs [67] , [68] . Similarly, thermal stability of COF- DhaTab samples synthesized at different time intervals (12, 24, 48 and 72 h) was monitored using TGA analysis under N 2 atmosphere, and shows almost identical behaviour (stable up to 350 °C). In order to find out the exact mechanism of the hollow sphere formation, we have analysed the COF- DhaTab samples isolated after 12, 24, 36, 48 and 72 h reaction time using TEM, SEM and AFM imaging ( Supplementary Figs 34–36 ). TEM images of the 12-h sample show rod-shaped morphology having lengths in the range 100–150 nm and width in the range 50 nm ( Fig. 3b and Supplementary Fig. 34 ). These crystallites are formed by the π–π stacking of COF layers along the c axis, as we have understood from the simulated crystal structure ( Fig. 3a ). The hexagonal pores of the DhaTab with regular pore channels in the crystallites can be viewed along the a and b axes ( Fig.3b ). As the reaction progresses, these crystallites are self-assembled into various shapes, including coiled and dense spherical structures ( Fig. 3b and Supplementary Fig. 22 ). After 24 h, the aggregation of the crystallites becomes more prominent and the morphology becomes more spherical ( Fig. 3b and Supplementary Fig. 34 ). However, the individual crystallites, which serve as the building units of the hollow spheres, can be clearly seen at the sphere walls under higher magnification. TEM images recorded for COF- DhaTab after a reaction time of 36 h shows the formation of hollow cavities inside the solid spheres ( Supplementary Fig. 34 ). As mentioned earlier, this happens as a result of inside-out Ostwald ripening [34] , [36] . The identical PXRD patterns of the COF- DhaTab samples isolated at different time intervals (12, 24, 36, 48 and 72 h) show high crystalline nature ( Fig. 2f ), which indicates that the self-assembly and the Ostwald ripening process of the crystallites do not perturb the internal ordering in the COF. Although the phenomenon of Ostwald ripening was well explained as a cause of hollow sphere formation in inorganic metal oxides [34] , [36] , in organic and polymer-based hollow spheres this phenomenon is rarely seen, since most of them are amorphous in nature. The purpose of inside-out Ostwald ripening was to minimize surface energy of the system. The crystallites in the inner part of the sphere have higher surface energy compared with the crystallite in the outer surface, since they have got higher curvature, being arranged in spheres of smaller radius [20] . To minimize the surface energy, crystallites redissolve [21] or migrate from the inner core and get recrystallized/self-assembled at the outer walls of the spheres. However, the wall of the hollow sphere formed at 36 h is not smooth, and the rod-like crystallite projections can be seen in the TEM image under higher magnification ( Fig. 3b and Supplementary Fig. 34 ). The TEM images recorded at 48 and 72 h show hollow spherical COF- DhaTab with a smooth sphere surface, which may have happened because of the fusion of the crystallites. Since the crystallite surface contains end functional groups (amine or aldehyde), they can undergo a Schiff base reaction leading to the formation of a smooth sphere wall surface. As mentioned already, the crystallinity and PXRD peak intensity of COF- DhaTab samples, isolated after the 12-h reaction time, remain identical. This shows that crystallization and growth of the COF- DhaTab crystallites are complete within a shorter reaction time (12 h) and after that self-assembly of the crystallites occurs, which finally leads to the unprecedented phenomenon of this chemically stable COF hollow sphere formation. This observation was supported by the TEM images at different time intervals: it was found that the size of COF crystallites synthesized at 24 and 36 h remains almost identical to that of the 12-h sample. However, a small decrease (4%) in surface area was observed for the COF- DhaTab synthesized at 72 h compared with the 12-h sample. We speculate that this change may be probably because of the fusion of the crystallite after 72 h. FT-IR, 13 C CP-MAS and TGA analyses of the COF- DhaTab sample isolated at different time show identical nature, indicating that chemical compositions are the same for 12- and 72-h COF samples ( Supplementary Figs 37–39 ). In order to understand the effect of reaction conditions on the evolution of the hollow spheres, we have synthesized the COF- DhaTab in different solvent combinations such as (a) mesitylene:dioxane—1:1, (b) mesitylene:dioxane—1.3:0.7, (c) mesitylene:dioxane—1.7:0.3, (d) mesitylene:dioxane—2:0 and at different temperature (80, 100 and 120 °C). From the TEM images it was understood that hollow sphere formation is more favourable in low concentrations of the dioxane (mesitylene:dioxane—2:0 and 1.7:0.3). When the concentration of dioxane increases (at mesitylene:dioxane—1.3:0.7 and 1:1) the count of hollow spheres observed in the sample starts decreasing and with distorted spherical morphology ( Supplementary Figs 40 and 41 ). The possible reason for this phenomenon is the water in oil-type behaviour of mesitylene:dioxane—2:0 or 1.7:0.3 system. TEM images of the COF-DhaTab sample synthesized at three different temperatures (80, 100 and 120 °C) show the hollow sphere formation. However, at 80 °C, along with hollow spheres some dense spherical structures were also observed ( Supplementary Fig. 42 ). To check the generality of hollow sphere formation on other COF systems, we have synthesized three reported keto-enamine-based COF ( COF-TpPa-1 (ref. 49 ), COF-TpBD [50] , COF-TpPa-F 4 (ref. 17 )) under the same reaction conditions of COF- DhaTab (mesitylene:dioxane:AcOH—1.7:0.3:0.2 at 120 °C). Interestingly, we were able to observe the formation of hollow spheres of COFs in the SEM images ( Supplementary Fig. 43 ). We also tried to synthesize a new imine-based COF ( DhaBad ) by using starting materials 2,5- Dha and Bad in mesitylene:dioxane (1.7:0.3 ml ) solvent combination. In this case hollow spheres were formed by the self-assembly of the microspheres ( Supplementary Fig. 6 ). We have investigated the mechanism of hollow sphere formation in DhaBad at different time intervals (12, 36 and 72 h). It was found that in the initial 12 h, DhaBad were evolved as particles of spherical morphology. As the time progresses, these small spheres self-assemble into various shapes such as fibres and particles with curved surface and so on (36 h). At 72 h, complete hollow sphere formation was observed ( Supplementary Fig. 44 ). Figure 3: Mechanism of hollow sphere formation. ( a ) Proposed mechanism of the formation of COF hollow spheres. ( b , c ) TEM and AFM images of COF- DhaTab , respectively, recorded at different intervals of time. Scale bars, ( b ) 12 h (200 nm, 100 nm), 24 h (100 nm, 50 nm), 36 h (200 nm, 50 nm), 72 h (200 nm, 20 nm) and ( c ) 12 h (500 nm), 24 h (500 nm), 36 h (100 nm), 72 h (100 nm). Full size image Enzyme adsorption Immobilization of enzymes in mesoporous materials is an important research area in biomedical and pharmaceutical industries [45] , [46] , [47] . The immobilization process not only improves the recyclability of the costly enzyme, but most of the time it can improve the stability of the enzyme under extreme conditions [48] . Microporous materials are not good choices for the enzyme immobilization as their pore sizes are too small to fit such large-sized biomolecules. Since COF- DhaTab is mesoporous in nature and has chemical stability in phosphate buffer and water, we have performed trypsin adsorption studies in it. Trypsin is a globular protein having hydrodynamic size of ∼ 3.8 nm, which is close to the COF- DhaTab pore size (3.7 Å). This close match in the relative size does not affect the trypsin adsorption in COF pores, since enzymes are soft molecules and can adjust their conformation to fit inside the COF pores ( Supplementary Fig. 45 ) [69] . The amount of trypsin absorbed in COF- DhaTab was estimated to be 15.5 μmol g −1 from the absorbance of residual unabsorbed trypsin in the decanted solution ( Supplementary Fig. 46 , Supplementary Methods ). In order to prove the enzyme adsorption inside the mesopores of COF- DhaTab , we have recorded the PXRD of the enzyme-loaded samples ( Fig. 4a ). It was found that the PXRD peak intensity gradually decreases as the amount of enzyme adsorption in the COF increases. This indicates the presence of enzyme inside the pores of COF, which will decrease the contrast intensity between COF walls and the empty pores. As a result, the peak intensity of the PXRD pattern decreases [48] . N 2 adsorption measurement of the trypsin-loaded COF- DhaTab sample shows a decrease in the BET surface area value (from 1,480 to 400 m 2 g −1 ), which also supports the immobilization of trypsin in COF pores ( Fig. 4c ). Successful immobilization of trypsin was confirmed by the confocal laser scanning microscopy (CLSM) of the fluorescein-labelled trypsin-loaded COF- DhaTab . The CLSM images show that the trypsin adsorption happens in the mesoporous walls of the hollow spheres and not in the macroscopic inner hollow cavity of the sphere ( Fig. 4g ). While moving from sphere wall to the centre of the hollow sphere, fluorescent intensity gets decreased considerably ( Supplementary Figs 47 and 48 ), which indicates that the inner part of the hollow sphere contains a very small amount of enzyme. The interaction between the nanometre (3.8 nm)-sized enzyme and the micrometer-sized inner voids is not feasible, as there is a large difference in the size ratio of the guest and the host. However, the inner empty space in the hollow spheres can provide a greater area of interaction sites for the incoming analyte molecules. TEM images of the trypsin-loaded samples show that the hollow sphere morphology remains intact even after the loading process ( Fig. 4e,f ). The retention of enzymatic activity after the immobilization of enzyme is an important feature, since in many cases after the immobilization process the enzyme loses its activity, either due to conformational change or by the hindrance of the catalytically active site. In order to find out the enzymatic activity of the trypsin-loaded COF- DhaTab, the sample was treated with 2 mM N-Benzoyl- L -arginine 4-nitroanilide in tris buffer (50 mM, pH 8) for 30 min. The visual colour change from colourless to yellow (due to the hydrolysis of N-Benzoyl-L-arginine 4-nitroanilide to p -nitroaniline) indicates that the activity of the enzyme was retained in the trypsin-loaded COF- DhaTab and the activity was found out to be 56.5 mmol g −1 min −1 ( Supplementary Figs 49 and 50 , Supplementary Methods ), which is ∼ 60% of the activity of the free enzyme. The enzyme-loading capacity of the COF- DhaTab and the catalytic activity of the enzyme-loaded COF is comparable to other literature-reported values ( Supplementary Tables 6 and 7 ). In addition to this, in the COF hollow sphere, we have performed the loading and release study of the anticancer drug doxorubicin (DOX). The amount of DOX loaded in COF was calculated as 0.35 mg g −1 ( Supplementary Figs 51 and 52 ). The drug release profile shows a slow release of DOX (42%) after 7 days in phosphate (pH 5) buffer ( Supplementary Fig. 53 ). This result indicates the potential of using the COF hollow sphere for the reversible binding and release of drug molecules. Figure 4: Trypsin loading in COF-DhaTab. ( a ) Schematic representation of trypsin adsorption in COF- DhaTab . ( b ) Amount of trypsin loading in COF- DhaTab at different solution concentration (the error bars represent the s.d. from triplicate measurements). ( c ) PXRD patterns of DhaTab after the adsorption of trypsin. ( d ) Comparison of N 2 adsorption isotherms DhaTab before and after trypsin loading. ( e ) TEM image of DhaTab ( e ) before and ( f ) after enzyme adsorption. ( g ) Confocal Z stacks of sections of fluorescein-labelled trysin-loaded single COF-DhaTab hollow sphere. Scale bars, ( e ) 100 nm, ( f ) 100 nm and ( g ) 2 μm. Full size image In summary, we have successfully synthesized chemically stable COF hollow spheres having mesoporous walls. The mechanism of hollow sphere formation was studied at different time intervals. We have rationalized that a self-assembly induced Ostwald ripening is responsible for the hollow sphere formation. The synthesized COF- DhaTab is highly crystalline and possesses high surface area of ∼ 1,500 m 2 g −1 . The presence of strong intramolecular H-bonding makes the COF structure rigid and flat, which is the reason behind the high surface area and crystallinity. This intramolecular H-bonding within the COF also enhances the hydrolytic stability. We have utilized the mesopores of COF- DhaTab for the immobilization of the enzyme trypsin. The maximum storage capacity of the trypsin for DhaTab was found to be 15.5 μmol g −1 . These results could lead to an initiation of the detailed investigation of COF crystallite formation and their self-assembly. We believe that the macroscopic pores inside the hollow spherical COF- DhaTab can provide greater number of interaction sites for the incoming analyte molecules to interact with the enzyme. Further investigations of this enzyme-immobilized COF as biosensor and biocatalyst is under progress. Isoreticulation of the mesoporous COFs with intramolecular hydrogen bonding sites, and their size-selective enzyme adsorption studies, are also under investigation. General information Complete details of the experimental and theoretical procedures are provided in the Supplementary Methods . 2,5- Dha was synthesized by 1,4-dimethoxybenzene according to a previously published procedure [70] . PXRD patterns were recorded on a Rigaku, MicroMax-007HF with high-intensity Microfocus rotating anode X-ray generator. All the samples were recorded in the 2 θ range of 2–40 degrees, and data were collected with the help of the Control Win software. A Rigaku, R axis IV++ detector was employed in wide-angle experiments. The radiation used was CuK (1.54 Å) with a Ni filter, and the data collection was carried out using an Aluminium holder. FT-IR spectra were taken on a Bruker Optics ALPHA-E spectrometer with a universal Zn-Se ATR (attenuated total reflection) accessory in the 600–4,000 cm –1 region or using a Diamond ATR (Golden Gate). TGA were carried out on a TG50 analyzer (Mettler-Toledo) or a SDT Q600 TG-DTA analyzer under N 2 atmosphere at a heating rate of 10 °C min –1 within a temperature range of 30–900 °C. SEM images were obtained with a Zeiss DSM 950 SEM and FEI, QUANTA 200 3D Scanning Electron Microscope with tungsten filament as electron source operated at 10 kV. The samples were sputtered with Au (nano-sized film) before imaging using a SCD 040 Balzers Union. TEM images were recorded using FEI Tecnai G2 F20 X-TWIN TEM at an accelerating voltage of 200 kV. The TEM samples were prepared by drop-casting the sample from isopropanol on copper grids TEM Window (TED PELLA Inc, 200 mesh). All gas adsorption experiments (up to 1 bar) were performed on a Quantachrome Quadrasorb automatic volumetric instrument. Solid-state NMR was taken in a Bruker 300 MHz NMR spectrometer and Ligand NMR data were taken in Bruker 300-MHz NMR spectrometer. CLSM images were taken with Carl Zeiss confocal system equipped with a 20 × objective. Synthesis of COF-DhaTab A pyrex tube (outside diameter (o.d.) × inner diameter (i.d. )=12 × 10 mm 2 and length 18 cm) is charged with Dha (21.6 mg; 0.13 mmol) and Tab (30.2 mg; 0.09 mmol), 1.7 ml of mesitylene, 0.3 ml of dioxane and 0.2 ml of 8.0 M aqueous acetic acid. This mixture was sonicated for 10 min in order to get a homogenous dispersion. The tube was then flash-frozen at 77 K (liquid N 2 bath) and degassed by three freeze-pump-thaw cycles. The tube was sealed off and then heated at 120 °C for 3 days. A yellowish orange-coloured precipitate formed was collected by centrifugation or filtration and washed with DMAc, water and then with ethanol. The powder collected was then solvent-exchanged with ethanol three times and then dried at 150 °C under vacuum for 24 h to give a yellowish orange-coloured powder in 80% (89 mg) isolated yield. IR (powder, ATR): 1,613, 1,588, 1,501, 1,442, 1,393, 1,335, 1,319, 1,212, 1,152, 1,012, 976, 885, 825, 767, 723, 621. For (C 12 H 8 NO) n ( DhaTab ), the elemental analysis (%) calcd. : C (79.11), H (4.43), N (7.69); found: C (79.68), H (4.45), N (7.42). Synthesis of COF DhaBad A pyrex tube (o.d. × i.d.=12 × 10 mm 2 and length 18 cm) is charged with Dha (21.6 mg; 0.13 mmol) and Bad (26.1 mg; 0.09 mmol), 1.7 ml of mesitylene, 0.3 ml of dioxane and 0.2 ml of 8.0 M aqueous acetic acid. This mixture was sonicated for 10 min in order to get a homogenous dispersion. The tube was then flash-frozen at 77 K (liquid N 2 bath) and degassed by three freeze-pump-thaw cycles. The tube was sealed off and then heated at 120 °C for 3 days. A yellowish orange-coloured precipitate formed was collected by centrifugation or filtration and washed with DMAc, water and then with ethanol. The powder collected was then solvent-exchanged with ethanol three times and then dried at 150 °C under vacuum for 24 h to give a yellowish orange-coloured powder in 85% (40 mg) isolated yield. IR (powder, ATR): 1,607, 1,495, 1,318, 1,277, 1,210, 1,154, 1,015, 967, 879, 830, 775, 725, 626. Elemental analysis (%) calcd. for (C 30 H 21 N 4 O 3 ) n ( DhaBad ): C (74.21), H (4.36), N (11.54), found C (73.42), H (4.21), N (11.37). Synthesis of COF-DhaTab at different time intervals COF reaction tubes were removed from the oven at different intervals of time (12, 24, 36, 48 and 72 h). After reaching room temperature, the reaction tube was broken and COF powders were thoroughly washed with DMAc, water and ethanol to remove any unreacted starting materials or polymeric side products ( Supplementary Table 8 ). The dry powdered samples of DhaTab were used as such for characterization with PXRD, TGA, FT-IR, and so on. For TEM, SEM and AFM imaging, 1 mg of DhaTab in 5 ml of isopropanol was sonicated for 10 min and subsequently coated on the carbon-coated copper grid (TEM) and Si-wafer or mica (AFM), and dried at room temperature before imaging. Loading of trypsin in COF-DhaTab For the loading studies, 2 mg of the COF- DhaTab was first sonicated in 2 ml of the phosphate buffer for 10 min in order to get a homogeneous dispersion. This buffer solution was degassed three times and treated with 2 mg of trypsin and stirred at 4 °C for 24 h in order to absorb the enzyme into the pores of the COF. After 24 h the solution was centrifuged and the absorbance of the decanted solution was noted using UV–vis spectrometer. Accession codes: The X-ray crystallographic coordinates for structures reported in this article have been deposited at the Cambridge Crystallographic Data Centre (CCDC), under deposition number CCDC 1010064. These data can be obtained free of charge from the Cambridge Crystallographic Data Centre via http://www.ccdc.cam.ac.uk/data_request/cif . How to cite this article: Kandambeth, S. et al. Self-templated chemically stable hollow spherical covalent organic framework. Nat. Commun. 6:6786 doi: 10.1038/ncomms7786 (2015).